Powering the programmed nanostructure and function of gold nanoparticles with catenated DNA machines DNA nanotechnology is a rapidly developing research area in nanoscience. It includes the development of DNA machines, tailoring of DNA nanostructures, application of DNA nanostructures for computing, and more. Different DNA machines were reported in the past and DNA-guided assembly of nanoparticles represents an active research effort in DNA nanotechnology. Several DNA-dictated nanoparticle structures were reported, including a tetrahedron, a triangle or linear nanoengineered nanoparticle structures; however, the programmed, dynamic reversible switching of nanoparticle structures and, particularly, the dictated switchable functions emerging from the nanostructures, are missing elements in DNA nanotechnology. Here we introduce DNA catenane systems (interlocked DNA rings) as molecular DNA machines for the programmed, reversible and switchable arrangement of different-sized gold nanoparticles. We further demonstrate that the machine-powered gold nanoparticle structures reveal unique emerging switchable spectroscopic features, such as plasmonic coupling or surface-enhanced fluorescence. The information encoded in the base-sequence of DNA attracts growing interest in designing functional DNA structures, and particularly DNA machines [1] , [2] , [3] . DNA machines performing ‘tweezers’ [4] , [5] , ‘walkers’ [6] , [7] , [8] , a ‘stepper’ [8] and more [9] mechanical functions, were reported. Different applications of DNA machines were suggested, including the transport of nanoparticles (NPs) on origami patterns [10] , the use of DNA nanomachines as logic gate devices [11] , [12] , and the application of molecular constructs in nanomedicine [13] . Also, self-organization of metal or semiconductor NPs, by means of DNA, into nanoengineered structures, attracts substantial recent interest, and ordered assemblies of variable geometries (linear, triangle and tetrahedron), which include dictated numbers and sizes of NPs, were reported [14] , [15] , [16] , [17] . Such nanoscale-engineered NP systems are anticipated to reveal unique plasmonic features such as interparticle plasmonic coupling [18] , [19] , [20] , [21] , [22] , chiroplasmonic properties [23] , [24] and surface-enhanced spectral functions, such as surface-enhanced Raman spectroscopy [25] or surface-enhanced fluorescence (SEF) [26] , [27] . Recent efforts are directed to the dynamic and programmed interconversion of NP architectures, particularly, the transition between two different configurations of the NPs [28] , [29] , [30] , [31] , [32] , [33] . Here, we demonstrate the dynamic and fuel-driven mechanical interconversion of a three-ring catenated nanostructure that enables the formation of structurally dictated and programmed NP assemblies. Photoswitchable plasmonic functions, such as interparticle plasmon coupling or SEF, are controlled by the NP-modified catenated DNA machine. Important future applications of such systems in nanomedicine and intracellular diagnostics may be anticipated [34] . Catenanes are interlocked, non-separable, ring systems and molecular catenanes were extensively used as molecular machines [35] . Synthesis and structural characterization of DNA catenanes have been reported [36] , [37] , [38] . Specifically, we have recently reported on the preparation of a three-ring catenane system, and the dynamic, reversible and switchable structural interconversion of the three-ring catenane system across three different ring configurations was demonstrated [39] . We now use the three-ring catenane system as a carrier for Au NPs (different sizes and dictated number of NPs). Microscopic characterization of programmed Au NP structures The Au NPs were functionalized with one or two nucleic acids (for the DNA sequences, synthesis and purification of the three-ring catenane and NPs, see Supplementary Table S1 and Supplementary Figs S1–S4 ). 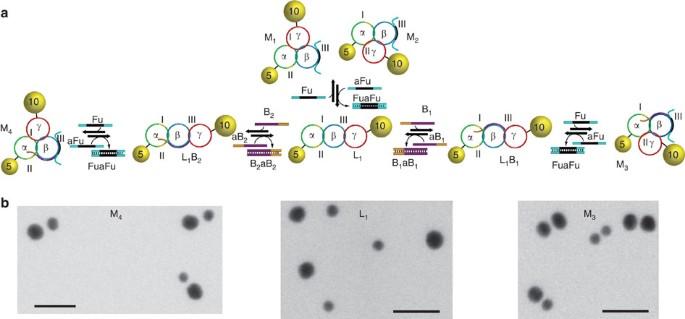Figure 1: Programmed assembly of two Au NPs structures. (a) Programmed structures of 5-nm and 10-nm Au NPs. (b) STEM images corresponding to the different Au NPs structures. Bars for the different images: 20 nm. Figure 1a shows the control of the interparticle distances between two Au NPs (5 and 10 nm) using a three-ring catenane machine. The 5-nm Au NP is hybridized to ring α, whereas the 10-nm NP is hybridized to ring γ to yield structure L 1 . The STEM image of the structure reveals an interparticle distance corresponding to 10.5±0.5 nm ( Fig. 1b ; for the respective histograms, see Supplementary Fig. S5a ). Ring α includes two equivalent domains, I and II, that are complementary to the domain III of ring γ. While the initial duplex between rings β and γ in region III is energetically favored, treatment of the ‘linear’ catenated system L 1 with a fuel strand (Fu) displaces ring γ that translocates, through hybridization, to either sites I or II of ring α (structures M 1 or M 2 ). In the presence of appropriate blocker units, the dictated directional translocation of ring γ, carrying the 10-nm Au NP, proceeds below or above the central ring β to yield the configurations M 3 or M 4 , respectively. The STEM image of the two NP configuration M 3 reveals an interparticle distance of 1.0±0.1 nm ( Supplementary Fig. S5b ), whereas the interparticle distance in configuration M 4 corresponds to 1.1±0.1 nm (for the respective histograms, see Supplementary Fig. S5c for an AFM image of the three-ring catenane associated with a single 5 nm NP, and for additional STEM images, refer to Supplementary Figs S6–S9 ). The interconversion across the three configurations is reversible and switchable. By addition of the appropriate anti-fuel and anti-blocker strands to the structures M 3 or M 4 , the structure L 1 is restored and it can be redirected to structure M 4 or M 3 , respectively. Upon analyzing several particle domains, through STEM characterization, we estimated the yield of the linear two NP structure to be 70%, and the conversion yield of structure L 1 to M 3 (or M 4 ) to be 80% (the conversion yield corresponds to ((M 3 or M 4 )/(L 1 +M 3 +M 4 )) × 100%; also, Supplementary Figs S10–S12 present STEM images of large areas of the two-NP assembly). While the interparticle distances in the three nanostructures L 1 , M 3 and M 4 follow the geometrical features of the assemblies, the precision of interparticle distances should be considered with caution. The flexibility of the single-stranded domains in the structures, drying effects of the nanostructures on the grid, the non-uniformity of the NP sizes (for the 5 nm, 5.4±0.9 nm; for the 10 nm, 8.1±1.1 nm) and the possible tethering of the NPs at in-plane/out-of-plane configurations, lead to distributions in the interparticle distances. Figure 1: Programmed assembly of two Au NPs structures. ( a ) Programmed structures of 5-nm and 10-nm Au NPs. ( b ) STEM images corresponding to the different Au NPs structures. Bars for the different images: 20 nm. Full size image The three-ring catenane system was further used as a machine for the dictated programmed assembly of Au NP structures of enhanced complexity by increasing the number of Au NPs associated with the catenated template. 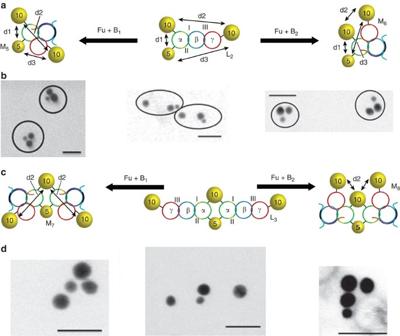Figure 2: Programmed organization of three and four Au NPs structures. (a) Programmed three NPs structures (1 × 5 nm; 2 × 10 nm). (b) STEMimages of the Au NPs structures generated by the DNA machine. (c) Programmed four Au NPs structures (1 × 5 nm; 3 × 10 nm) using the bis-three-ring catenane machine. (d) STEM images of the NPs structures generated by the cross-linked bis-three-ring catenane machine. Bars for thedifferent images: 25 nm. Figure 2a depicts the catenane machine-programmed organization of three different structures consisting of one 5-nm-sized Au NP and two 10-nm-sized Au NPs. In the quasilinear structure L 2 , the ring α is decorated with the 10-nm- and 5-nm-sized NPs, while the ring γ is functionalized with the 10-nm Au NP. In the presence of the respective blocker unit and Fu, the structures M 5 or M 6 are formed, respectively. Figure 2b shows the STEM images of the resulting machine-controlled Au NP structures. Three different interparticle distances d1, d2 and d3 characterize the structures. For the structure L 2 , the distances separating the respective Au NPs: d1, d2 and d3 correspond to 1.5±0.1, 14.6±0.4 and 10.1±0.4 nm, respectively (the histograms corresponding to the evaluation of the distances d1, d2 and d3 are shown in Supplementary Figure S13 . Also, for additional STEM images of the three different nanostructures, see Supplementary Figs S14–S16 ). The machine-induced formation of structure M 5 results in interparticle distances d1, d2 and d3: 1.1±0.1, 1.3±0.1 and 1.3±0.1 nm, respectively. In turn, the structure M 6 shows interparticle distances d1, d2 and d3: 1.1±0.1, 1.3±0.1 and 7.2±0.3 nm, respectively (the histograms corresponding to the evaluation of the distances are provided in Supplementary Figs S17 and S18 ). Analysis of large and different areas of the STEM grids indicated that the yield of the three Au NPs structure is 40% ( Supplementary Figs S19–S21 ). The rest of the nanostructures includes either two or single Au NPs. By analyzing large areas of the nanostructures and their respective characteristic d1, d2 and d3 distances, we estimated the yield of the translocation of L 2 to M 5 , or M 6 , to be ca. 70%, and the ‘purity’ of the M 5 or M 6 to be >90%. Figure 2c depicts the programmed organization of a four-Au NP structure (1 × 5 nm; 3 × 10 nm) using two interlinked three-ring catenane systems. The two three-ring catenanes are interlinked by a 5-nm Au NP and a 10-nm Au NP, each functionalized with two nucleic acids as hybridization tethers, for their dictated linkage to the respective domains within ring α. The rings γ in the bis-three-ring catenanes are each modified with a single nucleic acid-functionalized 10-nm-sized Au NP. This results in the structure L 3 as the parent nanostructure. The STEM images of structure L 3 , and the mechanically translocated structures M 7 and M 8 , confirm the formation of the programmed nanostructure. Upon using the appropriate blocker and upon moving ring γ through the bottom rim of ring β, by blocking its upper rim, structure M 7 is formed, and upon moving ring γ atop of ring β structure M 8 is formed (the blocker is hybridized to ring β on the bottom rim). The interparticle distances in the structures L 3 , M 7 and M 8 are similar to the distances observed for the analog parent structures L 2 , M 5 and M 6 (see Supplementary Figs S22, S23 and S24 ). Figure 2: Programmed organization of three and four Au NPs structures. ( a ) Programmed three NPs structures (1 × 5 nm; 2 × 10 nm). ( b ) STEMimages of the Au NPs structures generated by the DNA machine. ( c ) Programmed four Au NPs structures (1 × 5 nm; 3 × 10 nm) using the bis-three-ring catenane machine. ( d ) STEM images of the NPs structures generated by the cross-linked bis-three-ring catenane machine. Bars for thedifferent images: 25 nm. Full size image Controlled fluorescence by programmed Au NPs structures The dynamic mechanical positioning of different Au NPs on the catenane scaffold enabled us to control and switch plasmonic functions. Theoretical studies have addressed the effect of the proximity distance between a fluorophore and a Au NP of different sizes on the SEF/quenching process [26] , [27] . The SEF quantum yield in the presence of Au NPs is controlled by several parameters like the size of the Au NPs, the fluorophore quantum efficiency, the particles’ shape, the refractive index of the embedding medium, the distance separating the fluorophore and the Au NPs, and more. 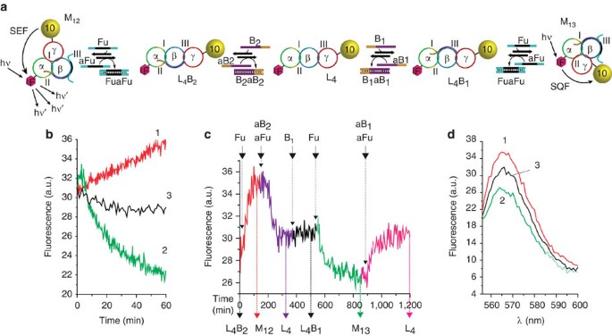Figure 3: Controlling the fluorescence properties of a dye/Au NP-functionalized DNA catenane machine. (a) Programmed switchable fluorescence properties of a dye associated with the three-ring catenane scaffold modified with a Au NP (10 nm). (b) Time-dependent fluorescence changes upon: (1) switching structure L4B2to M12(leading to SEF); (2) switching structure L4B1to M13(leading to SQF); (3) reaction of L4with Fu in the absence of blocker units to yield unblocked M12and M13. (c) Time-dependent normalized fluorescence changes upon the catenated DNA powered transition across the different states. Arrows on top indicate the time where the fuel/blocker, anti-fuel/anti-blocker strands are added, arrows at bottom indicate the state of the machine. (d) Fluorescence spectra corresponding to: (1) M12; (2) M13; (3) L4. Figure 3a depicts the switchable SEF/fluorescence quenching in the three-ring catenane machine modified with a fluorophore (Cy3)/Au NP (10 nm) pair. The fluorophore, F, is positioned close to site II of ring α, whereas the Au NP is positioned on ring γ to yield the linear structure L 4 . Figure 3b depicts the time-dependent fluorescence changes upon triggering the mechanical translocation in the three-ring catenane system. In the presence of the blocker hybridized to the lower rim of ring β, and upon addition of Fu that displaces ring γ, structure M 12 is formed. A time-dependent increase in the fluorescence of the dye is observed, suggesting that SEF proceeds (curve (1)). In turn, treatment of structure L 4 with a blocker that binds to the upper rim of ring β, and the addition of Fu, results in the translocation of ring γ to site II of ring α, bringing the fluorophore into close proximity to the Au NP, state M 13 . This results in the quenching of the fluorophore (curve (2)). Upon treatment of state L 4 with the Fu in the absence of any blocker unit, the negligible fluorescence changes depicted in curve (3) are observed, consistent with the similar probabilities to generate the two possible translocated states. The time-dependent fluorescence changes and the fluorescence spectra, across the different states of the molecular devices, are presented in Fig. 3c . Taking into account the different parameters affecting the fluorescence quantum yield of the specific fluorophore, in proximity to a 10-nm Au NP, we modeled the theoretical fluorescence intensity changes that are expected in the system ( Supplementary Fig. S25 and Supplementary Note 1 ; for an analysis of the reference quantum efficiency of Cy3, see Supplementary Table S2 ). The calculated results show that at a distance of 8 nm separating Cy3 from the 10-nm-sized Au NP, a ca. 20% increase in the fluorescence quantum yield is observed as compared with the reference fluorescence quantum yield. In turn, at a separating distance of <5 nm, the fluorophore undergoes quenching as compared with the fully separated NP–fluorophore system (configuration L 4 ). The computational results are consistent with the experimental data, showing enhanced fluorescence of structure M 12 (ca. 20%, increase in respect to the reference fluorescence, estimated separating distance of 7.3 nm) and enhanced quenching in structure M 13 (ca. 30%, estimated separating distance of 2.7 nm). Figure 3: Controlling the fluorescence properties of a dye/Au NP-functionalized DNA catenane machine. ( a ) Programmed switchable fluorescence properties of a dye associated with the three-ring catenane scaffold modified with a Au NP (10 nm). ( b ) Time-dependent fluorescence changes upon: (1) switching structure L 4 B 2 to M 12 (leading to SEF); (2) switching structure L 4 B 1 to M 13 (leading to SQF); (3) reaction of L 4 with Fu in the absence of blocker units to yield unblocked M 12 and M 13 . ( c ) Time-dependent normalized fluorescence changes upon the catenated DNA powered transition across the different states. Arrows on top indicate the time where the fuel/blocker, anti-fuel/anti-blocker strands are added, arrows at bottom indicate the state of the machine. ( d ) Fluorescence spectra corresponding to: (1) M 12 ; (2) M 13 ; (3) L 4 . Full size image Furthermore, positioning the fluorophore close to site I of ring α reverses the mechanical switchable fluorescence properties of the system (for the complete set of calculated distances, see Supplementary Table S3 ). Also, the fluorophore does not reveal any photobleaching within the time-scale of the experiments (see Supplementary Fig. S26 ). Controlled plasmonic interactions of Au NP structures We further examined the mechanically induced control of plasmonic coupling interactions in the different Au NP nanostructures generated by the DNA catenane machines. 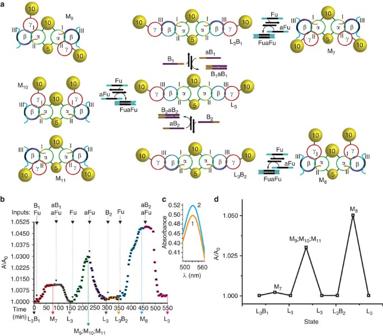Figure 4: Controlling the plasmonic properties of a Au NP nanostructure by a DNA catenane machine. (a) Reversible control of interparticle plasmonic interactions using a bis-three-ring catenane machine functionalized with four Au NPs (1 × 5 nm; 3 × 10 nm). (b) Time-dependent normalizedabsorbance changes upon the DNA machine-stimulated transition across the states. Arrows on top indicate the time where the fuel/blocker, anti-fuel/anti-blocker strands are added. (c) Absorbance spectra corresponding to: (1) L3B2state; (2) M8state. (d) Normalized absorbance values calculated according to the couple dipole theoretical model for the different states of the Au NPs shown in (a). Figure 4a exemplifies the different fuelled-programmed nanostructures generated by the bis-three-ring catenane machine that includes four Au NPs (3 × 10 nm Au NP+1 × 5 nm Au NP). Figure 4b shows the time-dependent normalized absorbance changes upon the programmed, fuel-driven transitions across the different NP structures. The treatment of the state L 3 B 1 with Fu results in structure M 7 , reflected by a low absorbance change. Treatment of the resulting structure with the anti-fuel and anti-blocker strands restores the structure L 3 . The subsequent treatment of structure L 3 with Fu (without any blocker) leads to a time-dependent absorbance increase as a result of the formation of the mixture of structures M 9 , M 10 and M 11 (2:1:1 ratio). The subsequent treatment of the mixture with anti-Fu, then, regenerates state L 3 . The interaction of L 3 with the blocker (B 2 ) and Fu leads to structure M 8 , characterized by a higher absorbance value, and treatment of state M 8 with the anti-blocker/anti-Fu restores the original absorbance of state L 3 , implying that the plasmonic interactions in the different structures are reversible. Figure 4c (curve (1)) shows the spectrum of the structure L 3 B 2 , whereas, Fig. 4c (curve (2)) gives the absorption spectra of nanostructures M 8 , after treatment of L 3 B 2 with Fu. This absorbance is reversible, and treatment of the resulting structure M 8 with the anti-fuel/anti-blocker strands restores the spectrum shown in curve (1) (For the detailed discussion of the time-dependent absorbance spectra and reversible switching between structures L 3 B 2 , M 8 and L 3 , see Supplementary Discussion ). The different plasmonic interactions can be attributed to the different sizes and geometrical distances separating the particles in the different assemblies (see Supplementary Figs S27–S30 ). Note that the rates of recovery of states L 3 from M 7 and M 8 or the mixture M 9 –M 10 –M 11 are different. While an induction period is required to restore L 3 from M 7 and M 8 , the regeneration of L 3 from the M 9 –M 10 –M 11 mixture does not involve an induction. This is due to the fact that the formation of L 3 from M 7 and M 8 involves a primary, slow displacement process of the blocker, while the formation of L 3 from the mixture M 9 –M 10 –M 11 does not include a deblocking reaction. As the spatial arrangement of the different-sized particles differ in structures L 3 , M 7 –M 9 , M 8 –M 10 and M 11 , the plasmonic absorbance of coupled particles should change in the respective structures. Particularly, in the systems M 8 and M 10 , the larger Au NPs (10 nm) retain a compact intimate configuration with strong interparticle plasmonic interactions, and thus the enhanced absorbance in these structures should prevail. The configurations M 11 and M 7 should also show a small degree of enhancement due to the relatively compact arrangements of the large Au NPs, whereas the state L 3 should have the least interaction and, correspondingly, noticeable enhancement of absorbance for such a state is not expected. It should be noted that the plasmonic absorbance changes are presented as a ratio A/A 0 , where A 0 is the absorbance of the reference linear nanostructure L 3 , and A is the absorbance of the respective dynamically generated Au NP nanostructures. Although the experimental system consists of a heterogeneous population composed, also, of ‘incomplete’ NP structures and contributions of ‘incorrect’ configurations of Au NPs, we find that this heterogeneous mixture of components has only a minute effect on the A/A 0 ratio (cf. A/A 0 of M 7 or of other configurations shown in Supplementary Fig. S31 ). Thus, the absorbance changes of the system, upon treatment of structure L 3 with B 2 and Fu, may be, mainly, attributed to the formation of the structure M 8 . Accordingly, the absorbance features of the configurations L 3 , M 7 –M 9 , M 8 –M 10 and M 11 were theoretically modeled using the coupled dipole method [20] , [21] , [22] ( Fig. 4d ; for further details, see Supplementary Note 2 ). In these calculations, we used the geometrically estimated distances separating the different particles in the respective configuration. We find that the calculated absorption features of the different NP configurations nicely follow the experimental results. It should be noted, moreover, that the observed absorbance changes upon the dynamic transitions across the configurations cannot originate from phenomena such as aggregation of the NPs. This phenomenon is neither observed in the STEM images nor visually observed through precipitation of the particles. Furthermore, the absorbance changes shown in Fig. 4b reach a saturation value that cannot be rationalized in terms of a continuous dynamic aggregation process. Simultaneously, Fig. 4b is consistent with the calculations based on the coupled plasmonic model. Figure 4: Controlling the plasmonic properties of a Au NP nanostructure by a DNA catenane machine. ( a ) Reversible control of interparticle plasmonic interactions using a bis-three-ring catenane machine functionalized with four Au NPs (1 × 5 nm; 3 × 10 nm). ( b ) Time-dependent normalizedabsorbance changes upon the DNA machine-stimulated transition across the states. Arrows on top indicate the time where the fuel/blocker, anti-fuel/anti-blocker strands are added. ( c ) Absorbance spectra corresponding to: (1) L 3 B 2 state; (2) M 8 state. ( d ) Normalized absorbance values calculated according to the couple dipole theoretical model for the different states of the Au NPs shown in ( a ). Full size image The present study has introduced a method to power the programmed organization of Au NP nanostructures using catenated DNA machines as templates. Our study has demonstrated that the mechanically driven, reversible transitions of a fluorophore/Au NP pair or a multi-Au NP system across dictated nanostructures leads to switchable and programmed SEF/fluorescence quenching phenomena and to structurally controlled interparticle plasmonic interactions. Specifically, we addressed the theoretical modeling of the interparticle plasmonic interactions between the different Au NP nanostructures, and the distance-dependent fluorescence quenching or fluorescence enhancement in the different Au NP/fluorophore configurations. We found very good agreement between the theoretical predictions and the experimental results. Thus, we suggest that similar theoretical modeling of the optical properties of Au NP nanostructures or Au NP/fluorophore hybrid systems should be an essential element in understanding the experimental photophysics of such nanostructures. This study paves the grounds to implement other DNA machines, for example, tweezers, to generate programmed dynamically reconfigurable structures of Au NPs or fluorophore/Au NP assemblies, exhibiting controlled plasmonic properties. By implementing different-sized NPs, and different metal NPs, a rich arena of plasmonic nanostructures for theoretical modeling is envisaged [40] . Synthesis and purification of the Au NP/DNA nanostructures Detailed protocols for the synthesis and purification of the three-ring DNA catenane and for the preparation of the DNA/Au NP conjugates and their purification, can be found in the Supplementary Methods . After mixing the Au NPs/DNA conjugates with the catenane scaffold, in the appropriate buffer solution, containing a high salt concentration, the DNA tethers were allowed to hybridize for 2 hours, at 25°C. After that, the different Au NP/three-ring DNA catenane systems were purified at 10 °C using agarose gel electrophoresis (MetaPhor, Lonza). The respective gel band was then excised, and the product extracted into a dialysis membrane (10 kDa MWCO, Snakeskin, Thermoscientific). The solution was, then, filtered through a 0.22-μm membrane (Whatman), and the nanostructures were collected using Amicon filtering tubes (100 kDa MWCO, Millipore). The Au NP/DNA/fluorophore nanostructure was prepared by mixing the DNA scaffold, the fluorophore modified nucleic acid and the single DNA strand-modified Au NPs in a 1:1:1 molar ratio. Operation of the different Au NP/DNA (Cy3) hybrid machines To activate the respective Au NP/DNA (Cy3) hybrid machines, an excess of the blocker/anti-blocker strands and the respective fuel/anti-fuel was added in the appropriate order to a high-salt concentration buffer solution (0.1 × TBE, 0.4 mg ml −1 bis (p-sulphonatophenyl) phenylphosphine dihydrate dipotassium salt, 700 mM NaCl) containing the Au NP/DNA machine 20 nM. The fluorescence analyses were performed with a Cary Eclipse Varian with an excitation wavelength of 540 nm and acquiring the emission at 560 nm wavelength. The experiments probing the plasmonic interactions were carried out with a Shimadzu UV-2401PC spectrophotometer, recording the absorbance at 520 nm. All operations were conducted at 25 °C. STEM pictures were taken with an extra high-resolution scanning electron microscope (Magellan 400L). The nanostructures for STEM analyses were prepared in the buffer solution already described above, and eventually diluted to a final concentration of 2 nM in a 200 mM NaCl solution. Detailed explanations of the experimental protocols are presented in the Supplementary Methods . J.E. and I.W. designed the project; J.E. and A.C. performed the experiments; Z.F. and A.O.G. provided the theoretical model for the dynamically controlled plasmonicinteractions of Au NP nanostructures; J.E., A.C. and I.W. wrote the paper. How to cite this article: Elbaz, J. et al . Powering the programmed nanostructure and function of gold nanoparticles with catenated DNA machines. Nat. Commun. 4:2000doi: 10.1038/ncomms3000 (2013).